Endoplasmic reticulum calcium release through ITPR2 channels leads to mitochondrial calcium accumulation and senescence Senescence is involved in various pathophysiological conditions. Besides loss of retinoblastoma and p53 pathways, little is known about other pathways involved in senescence. Here we identify two calcium channels; inositol 1,4,5-trisphosphate receptor, type 2 (ITPR2) (also known as inositol 1,4,5-triphosphate receptor 2 (IP3R2)) and mitochondrial calcium uniporter (MCU) as new senescence regulators in a loss-of-function genetic screen. We show that loss of ITPR2, known to mediate endoplasmic reticulum (ER) calcium release, as well as loss of MCU, necessary for mitochondrial calcium uptake, enable escape from oncogene-induced senescence (OIS). During OIS, ITPR2 triggers calcium release from the ER, followed by mitochondrial calcium accumulation through MCU channels. Mitochondrial calcium accumulation leads to a subsequent decrease in mitochondrial membrane potential, reactive oxygen species accumulation and senescence. This ER-mitochondria calcium transport is not restricted to OIS, but is also involved in replicative senescence. Our results show a functional role of calcium release by the ITPR2 channel and its subsequent accumulation in the mitochondria. Senescence is characterized by a stable proliferation arrest accompanied by the acquisition of several specific features. It is activated by numerous cellular stresses, such as replicative exhaustion, oncogenic signals or oxidative stress [1] . It is now accepted that senescence induction acts as a protective mechanism against oncogenic events, tumour initiation and progression [2] , [3] , [4] , [5] . Besides the cancer-regulated role of senescence, it is also known to be involved in an increasing number of other processes, such as wound healing and various aging-related diseases [6] , [7] . Most of the pathways known to regulate senescence and, in particular, senescence escape, point to a central role of the p53 as well as the p16–retinoblastoma pathways [8] . Nevertheless, emerging evidences support the existence of other mechanisms regulating senescence escape, although, to date, little is known about these mechanisms [9] , [10] , [11] , [12] , [13] , [14] , [15] . Most of the data demonstrating a central role of the p53 and its upstream activators (DNA damage, p14 ARF ) and p16 INK4A –retinoblastoma pathways were performed in fibroblasts. Similar data generated in human epithelial cells or in other lineages are rather rare, and display a more complex picture of the genetic events involved in senescence escape [15] . For example, human mammary epithelial cells (HECS), which are known to not express p16 INK4A (ref. 16 ), enter senescence in response to oncogenic stress in a DNA damage/p53-independent manner [14] , [15] . Here, we identify inositol 1,4,5-trisphosphate receptor, type 2 (ITPR2) and mitochondrial calcium uniporter (MCU) as two new actors of senescence, whose knockdown results in senescence escape. Their identification sheds light on the role of calcium movement, and in particular, mitochondrial calcium accumulation in senescence induction. Identification of calcium channels as senescence modulators To isolate new senescence regulators, we have performed a loss-of-function genetic screen covering the entire genome to isolate specific small-hairpin RNAs (shRNAs) allowing oncogene-induced senescence (OIS) escape in immortalized HECs. We used post-stasis HECs, which do not express p16 INK4A (ref. 16 ), immortalized by stable expression of hTert (HEC–telomerase reverse transcriptase (Tert)). Cells were infected to stably express MAPK/ERK kinase (MEK):endoplasmic reticulum (ER), a 4-hydroxytamoxifen (4OHT) inducible MEK oncogene, to induce oncogenic stress (HEC–TM). HEC–TM cells were treated with 4OHT at doses not affecting HEC-Tert cell growth. HEC–TM were infected with an shRNA library covering the whole genome and treated every 2 days with 4OHT to induce senescence. Cells having escaped senescence were amplified and their shRNA identified. We have identified multiple potential shRNA-targeted genes. Details of the screening strategy, methods and results were previously described in Lallet-Daher et al. [17] We were particularly interested in focusing our work on the ITPR2 calcium channel. This channel is a member of the inosotol 1,4,5-triphosphate (IP3) receptor (ITPR) family, composed of two other members: ITPR1 and ITPR3, the most ubiquitously expressed family of calcium-released channel of the ER. 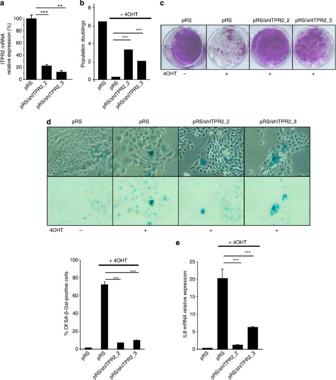Figure 1: ITPR2 knockdown promotes escape from OIS. HEC–TM cells were infected with a control empty vector (pRS) or with two independent ITPR2-targeting shRNA (shITRP2_2 and 3) retroviral vectors and then the selected puromycin. (a) RNAs were extracted, retro-transcribed and ITPR2 mRNA levels analyzed by quantitative PCR. ITPR2 mRNA expression was normalized to β-actin mRNA expression. (b) Cells were treated daily with 4OHT for 3 days to induce senescence. Six days after the 4OHT treatment, cells were counted and the number of population doublings was calculated. (c) After seeding, cells were treated daily with 4OHT for 3 days. After 10 days, cells were paraformaldehyde fixed and crystal violet stained to monitor cell growth. (d) Cells were seeded and 4OHT treated. Six days later, cells were fixed and SA-β-Gal activity was assayed (mean±s.d. are shown). (e) Cells were seeded and 4OHT treated. RNAs were extracted and expression of the IL8 senescence marker analyzed by RT–qPCR. IL8 mRNAs were normalized against β-actin levels. Images shown are representative of experiments performed at least three times. Graphs are presented with s.e.m. as errors bars, except for panel (d), and the studentt-test was used to determine theP-value. **P<0.01; ***P<0.001. A search in the Oncomine database, a cancer microarray database allowing differential expression analyses between the most major types of cancer and normal tissues, showed a general decrease of ITPR2 mRNA in numerous cancer types ( Supplementary Table 1 ) although an increase in ITPR2 mRNA was also observed in other cancer types ( Supplementary Table 1 ). Interestingly, in the majority of cases, this increase was detected in benign tumours such as oncocytoma ( Supplementary Fig. 1a ) and prostatic intraepithelial neoplasia ( Supplementary Fig. 1b ), benign tissues being known to accumulate senescent cells [3] . Finally, ITPR2 levels were found to be significantly lower in primary breast tumours in a cohort of patients displaying metastasis versus the metastasis-free group ( Supplementary Fig. 1c ). Together, these observations prompted us to study the role of ITPR2 in oncogene-induced senescence escape, a key step required for tumour initiation and progression. ITPR2 knockdown promotes OIS escape To validate the role of ITPR2 in OIS, we generated two different ITPR2-targeting shRNAs. As expected, these shRNA strongly decreased ITPR2 mRNA levels ( Fig. 1a ) without impacting ITPR1 and ITPR3 mRNA levels ( Supplementary Fig. 2a ). Functionally, ITPR2 depletion by these two shRNAs overcame the growth arrest induced by oncogenic stress (+4OHT), as measured by the ability of the cells to maintain their growth ( Fig. 1b,c ). Knockdown also resulted in a decrease of two independent senescence markers; senescence-associated beta-galactosidase (SA-β-Gal) activity ( Fig. 1d ) and interleukin 8 expression ( Fig. 1e ), further confirming a role of ITPR2 in OIS escape. By performing quantitative reverse transcriptase-PCR (qRT–PCR), we found that ITPR1, 2 and 3 were all expressed in HEC–TM cells ( Supplementary Fig. 2b ). Interestingly, ITPR1 ( Supplementary Fig. 2c ) and ITPR3 knockdown ( Supplementary Fig. 2d ), also promoted OIS escape ( Supplementary Fig. 2e ). Of note, expression of ITPR1, 2 and 3 were only slightly altered during senescence, suggesting their role during senescence might be owing to alterations of their activities rather than alteration of their expression ( Supplementary Fig. 2f ). Figure 1: ITPR2 knockdown promotes escape from OIS. HEC–TM cells were infected with a control empty vector (pRS) or with two independent ITPR2-targeting shRNA (shITRP2_2 and 3) retroviral vectors and then the selected puromycin. ( a ) RNAs were extracted, retro-transcribed and ITPR2 mRNA levels analyzed by quantitative PCR. ITPR2 mRNA expression was normalized to β-actin mRNA expression. ( b ) Cells were treated daily with 4OHT for 3 days to induce senescence. Six days after the 4OHT treatment, cells were counted and the number of population doublings was calculated. ( c ) After seeding, cells were treated daily with 4OHT for 3 days. After 10 days, cells were paraformaldehyde fixed and crystal violet stained to monitor cell growth. ( d ) Cells were seeded and 4OHT treated. Six days later, cells were fixed and SA-β-Gal activity was assayed (mean±s.d. are shown). ( e ) Cells were seeded and 4OHT treated. RNAs were extracted and expression of the IL8 senescence marker analyzed by RT–qPCR. IL8 mRNAs were normalized against β-actin levels. Images shown are representative of experiments performed at least three times. Graphs are presented with s.e.m. as errors bars, except for panel ( d ), and the student t -test was used to determine the P -value. ** P <0.01; *** P <0.001. Full size image IP3-induced ITPR activation induces premature senescence We next wanted to know whether a gain-of-function of ITPR activity affected senescence. To this end, the ITPR ligand, IP3 (membrane-permeant), was used to activate ITPR. Interestingly, ITPR activation blocked cell growth ( Fig. 2a,b ), induced SA-β-Gal activity ( Fig. 2c ) and the interleukin 8 senescence marker expression ( Fig. 2d ). Together, the data show that ITPR loss-of-function promotes OIS escape, whereas ITPR activation by IP3 induces a premature senescence. 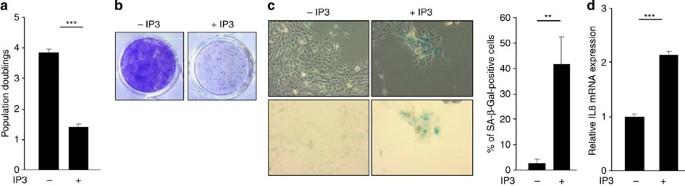Figure 2: ITPR activation induces premature senescence. HEC–TM cells were seeded at the same density and treated or not every day for 5 days with 5 μM IP3. The following day, various assays were performed. (a) Cells were counted and the number of population doublings was calculated. (b) Cells were paraformaldehyde fixed and crystal violet stained to monitor cell growth. (c) Cells were fixed and SA-β-Gal activity was assayed. Means±s.d. are presented in the graph. (d) RNAs were extracted and expression of the IL8 senescence marker analyzed by RT–qPCR. IL8 mRNAs were normalized to β-actin levels. Images shown are representative of experiments performed at least twice. Graphs are presented with s.e.m. as errors bars, except for panel (c), and the studentt-test was used to determine theP-value. **P<0.01; ***P<0.001. Figure 2: ITPR activation induces premature senescence. HEC–TM cells were seeded at the same density and treated or not every day for 5 days with 5 μM IP3. The following day, various assays were performed. ( a ) Cells were counted and the number of population doublings was calculated. ( b ) Cells were paraformaldehyde fixed and crystal violet stained to monitor cell growth. ( c ) Cells were fixed and SA-β-Gal activity was assayed. Means±s.d. are presented in the graph. ( d ) RNAs were extracted and expression of the IL8 senescence marker analyzed by RT–qPCR. IL8 mRNAs were normalized to β-actin levels. Images shown are representative of experiments performed at least twice. Graphs are presented with s.e.m. as errors bars, except for panel ( c ), and the student t -test was used to determine the P -value. ** P <0.01; *** P <0.001. Full size image Oncogene stress provokes mitochondrial calcium relocation As ITPR2 and the other members of ITPR family are calcium channels involved in regulating the exit of calcium from the ER [18] , we examined calcium changes during OIS using the Oregon Green calcium probe. We tracked calcium in live proliferating cells (−4OHT) and in cells in OIS (+4OHT). We observed a strong change in calcium localization and pattern as it accumulated in dots in the cytoplasm of senescent cells ( Fig. 3a,b ). Interestingly, a change in calcium pattern was not found in ITPR2-knockdown cells ( Fig. 3a,b ). We conclude that senescent cells, at least in response to oncogenic stress, display an altered calcium homoeostasis and this phenomena involves the ITPR2 channel. 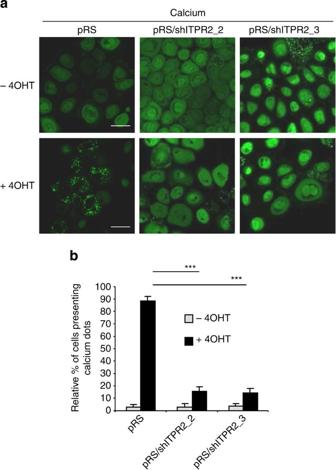Figure 3: ITPR2 participates in calcium movement during OIS. (a) HEC–TM cells expressing or not an shRNA directed against ITPR2 were seeded at the same density. The following day, they were treated daily with 4OHT for 3 days and the next day, living cells were incubated with the calcium probe (Oregon green) and their fluorescence analyzed by confocal microscopy. (b) Percentage of cells displaying calcium dots was calculated for each condition. Scale bar, 50 μM. Graphs are presented with s.e.m. as errors bars, and the studentt-test was used to determine theP-value. ***P<0.001. Figure 3: ITPR2 participates in calcium movement during OIS. ( a ) HEC–TM cells expressing or not an shRNA directed against ITPR2 were seeded at the same density. The following day, they were treated daily with 4OHT for 3 days and the next day, living cells were incubated with the calcium probe (Oregon green) and their fluorescence analyzed by confocal microscopy. ( b ) Percentage of cells displaying calcium dots was calculated for each condition. Scale bar, 50 μM. Graphs are presented with s.e.m. as errors bars, and the student t -test was used to determine the P -value. *** P <0.001. Full size image Oncogene stress lead to mitochondrial calcium accumulation We next wanted to determine the altered localization of calcium in senescent cells. We hypothesized that the mitochondria would be involved in this redistribution, since calcium release by the ER can be transferred to mitochondria [19] , and also because the MCU [20] , [21] , a key component in mitochondrial calcium uptake, was identified in the genetic screen [17] . To examine the localization of calcium dots in senescent cells, we used an red fluorescent protein (RFP)-tagged mitochondrial protein which showed that the calcium dots co-localize with the mitochondria during OIS ( Fig. 4a , yellow dots). To further confirm mitochondrial calcium accumulation in senescent cells, we introduced a genetically encoded, mitochondrially targeted calcium indicator ‘mito-GCaMP2’ (ref. 22 ). The specificity of this mitochondrial calcium reporter was demonstrated as its fluorescence increased following IP3 treatment, which was inhibited when the cells were pre-treated with an inhibitor of MCU (Ru360) ( Fig. 4b ). Importantly, we observed a fluorescence increase in senescent cells, absent in ITPR2-knockdown cells ( Fig. 4c ). Inversely, ITPR activation by IP3 treatment, which induced senescence ( Fig. 2 ), also resulted in mitochondrial calcium accumulation ( Fig. 4d ). Overall, this demonstrates that senescent cells accumulate calcium in mitochondria, with calcium accumulation and OIS being abolished in ITPR2-knockdown cells. 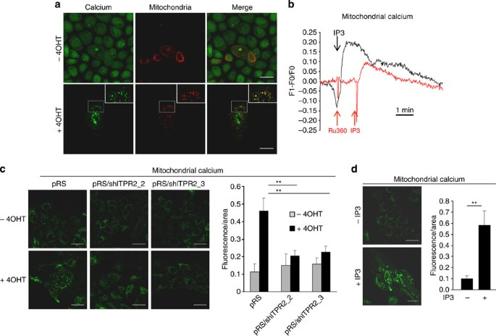Figure 4: Oncogenic stress induces mitochondrial calcium uptake during OIS. (a) HEC–TM cells were seeded at the same density, treated or not with 4OHT, transduced to express an RFP-coupled mitochondrial protein and a day later labelled by the calcium probe. Live cells fluorescence was examined using confocal microscopy. (b) HEC–TM cells were infected with a retroviral vector encoding the mitochondrial calcium genetic reporter (mito-GCaMP2). Cells were treated with 5 μM IP3, with or without 10 μM Ru360 MCU inhibitor. Fluorescence intensities in at least five ROI were recorded and results displayed. (c) Senescence was induced by 4OHT treatment for 3 days. Three days after the end of this treatment, mitochondrial calcium reporter fluorescence intensity was recorded and quantified for each condition (n>5 fields for nontreated cells,n>10 fields for treated cells). Quantification is representative of experiments performed at least three times. (d) Cells were treated or not with 5 μM IP3 for 5 days. The following day, mitochondrial calcium reporter fluorescence intensity was recorded and quantified for each condition (n>15 fields). Scale bar, 50 μM. Graphs are presented with s.e.m. as errors bars, and the studentt-test was used to determine theP-value. **P<0.01. Figure 4: Oncogenic stress induces mitochondrial calcium uptake during OIS. ( a ) HEC–TM cells were seeded at the same density, treated or not with 4OHT, transduced to express an RFP-coupled mitochondrial protein and a day later labelled by the calcium probe. Live cells fluorescence was examined using confocal microscopy. ( b ) HEC–TM cells were infected with a retroviral vector encoding the mitochondrial calcium genetic reporter (mito-GCaMP2). Cells were treated with 5 μM IP3, with or without 10 μM Ru360 MCU inhibitor. Fluorescence intensities in at least five ROI were recorded and results displayed. ( c ) Senescence was induced by 4OHT treatment for 3 days. Three days after the end of this treatment, mitochondrial calcium reporter fluorescence intensity was recorded and quantified for each condition ( n >5 fields for nontreated cells, n >10 fields for treated cells). Quantification is representative of experiments performed at least three times. ( d ) Cells were treated or not with 5 μM IP3 for 5 days. The following day, mitochondrial calcium reporter fluorescence intensity was recorded and quantified for each condition ( n >15 fields). Scale bar, 50 μM. Graphs are presented with s.e.m. as errors bars, and the student t -test was used to determine the P -value. ** P <0.01. Full size image Mitochondrial calcium accumulation mediates OIS To functionally demonstrate that calcium entry is a key event in ITPR-mediating OIS, we performed knockdown against MCU. As expected, MCU-knockdown cells ( Fig. 5a ) displayed a strong decrease in mitochondrial calcium accumulation following oncogenic stress induction ( Fig. 5b ). This decreased mitochondrial calcium level allowed cells to escape OIS, as measured by their ability to proliferate ( Fig. 5c,d ) and the absence of senescence markers ( Fig. 5e,f ). In addition, knockdown of MICU1 ( Supplementary Fig. 3a ), an interactor and modulator of MCU [23] , [24] , potentiated low oncogenic stress to induce OIS ( Supplementary Fig. 3b,c ) with concomitant mitochondrial calcium accumulation ( Supplementary Fig. 3d ). 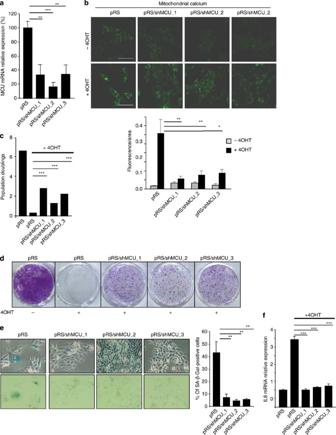Figure 5: MCU knockdown blocks mitochondrial calcium accumulation and induces OIS escape. HEC–TM cells were infected with a control empty vector (pRS) or independent MCU-targeting shRNA retroviral vectors and then puromycin selected. (a) RNA were prepared and retro-transcribed. Quantitative PCR against MCU was performed and the results were normalized to β-actin mRNA levels. (b) Cells transduced with a mitochondrial calcium genetic reporter were seeded at the same density, treated with 4OHT for 3 days. Four days later, fluorescence intensities were recorded and results displayed (n>5 fields for nontreated cells,n>10 fields for treated cells). (c) After seeding the same amount of cells, they were treated daily with 4OHT for 3 days to induce senescence. Six days after the 4OHT treatment, cells were counted and the number of population doublings was calculated. (d) Empty pRS or shRNA-MCU expressing cells were seeded at the same density, treated for 3 days with 4OHT. Ten days later, cells were paraformaldehyde fixed and crystal violet stained to monitor cell growth. (e) Cells were seeded, and treated for the next 3 days with 4OHT. Six days later, cells were fixed and an SA-β-Gal assay performed. SA-β-Gal-positive cells were counted and representative photographs are shown (Mean±s.d.) (f) The day after seeding, cells were 4OHT treated for 3 days. Two days later, RNAs were prepared, retro-transcribed and analyzed by quantitative PCR against IL8 and normalized to β-actin levels. Scale bar, 50 μM. Graphs are presented with s.e.m. as errors bars, except for panel (e), and the studentt-test was used to determine theP-value. *P<0.05; **P<0.01; ***P<0.001. Figure 5: MCU knockdown blocks mitochondrial calcium accumulation and induces OIS escape. HEC–TM cells were infected with a control empty vector (pRS) or independent MCU-targeting shRNA retroviral vectors and then puromycin selected. ( a ) RNA were prepared and retro-transcribed. Quantitative PCR against MCU was performed and the results were normalized to β-actin mRNA levels. ( b ) Cells transduced with a mitochondrial calcium genetic reporter were seeded at the same density, treated with 4OHT for 3 days. Four days later, fluorescence intensities were recorded and results displayed ( n >5 fields for nontreated cells, n >10 fields for treated cells). ( c ) After seeding the same amount of cells, they were treated daily with 4OHT for 3 days to induce senescence. Six days after the 4OHT treatment, cells were counted and the number of population doublings was calculated. ( d ) Empty pRS or shRNA-MCU expressing cells were seeded at the same density, treated for 3 days with 4OHT. Ten days later, cells were paraformaldehyde fixed and crystal violet stained to monitor cell growth. ( e ) Cells were seeded, and treated for the next 3 days with 4OHT. Six days later, cells were fixed and an SA-β-Gal assay performed. SA-β-Gal-positive cells were counted and representative photographs are shown (Mean±s.d.) ( f ) The day after seeding, cells were 4OHT treated for 3 days. Two days later, RNAs were prepared, retro-transcribed and analyzed by quantitative PCR against IL8 and normalized to β-actin levels. Scale bar, 50 μM. Graphs are presented with s.e.m. as errors bars, except for panel ( e ), and the student t -test was used to determine the P -value. * P <0.05; ** P <0.01; *** P <0.001. Full size image Our results support the findings that, during OIS, calcium released from the ER through ITPR channels accumulates in the mitochondria, resulting in senescence. An ER/mitochondria liaison can facilitate calcium exchange between both organelles [19] . We then examined ER/mitochondria contact sites by co-labelling both organelles and counting co-localized signals to examine whether there was any change during OIS. No changes in the number of contact sites were observed during OIS or in ITPR2-knockdown cells ( Supplementary Fig. 4 ). Mitochondrial calcium leads to mitochondrial potential drop The next question we wanted to address was how mitochondrial calcium overload leads to OIS. Abnormal levels of calcium in the mitochondria are known to result in a decrease of the mitochondrial potential (Δψ(m)) [25] , [26] . We observed a drop in the Δψ(m) during OIS, as assayed by the fluorescence intensity drop of the Rhodamine 123 ( Supplementary Fig. 5 ) and by the ratiometric change of JC-1 fluorescence ( Fig. 6a,b ). Oncogenic stress-induced mitochondrial depolarization was not observed in ITPR2- or MCU-knockdown cells ( Fig. 6a,b and Supplementary Fig. 5 ), suggesting that mitochondrial calcium overload during OIS triggers the Δψ(m) drop. This was largely supported by the observation that, following oncogenic stress induction, mitochondrial calcium accumulation occurred before the Δψ(m) drop ( Supplementary Fig. 6 ). While our results suggest that mitochondrial calcium accumulation is the initiating event and that it precedes depolarization, it is also probable that depolarization further amplifies mitochondrial calcium accumulation as previously described [27] . To assess the role of Δψ(m) drop during senescence, we treated cells with the carbonyl cyanide 4-(trifluoromethoxy)phenylhydrazone (FCCP)uncoupler to force mitochondrial depolarization ( Fig. 7a ). Mitochondrial depolarization was found to block cell growth ( Fig. 7b,c ) and to induce senescence markers ( Fig. 7d,e ) supporting a key role of a Δψ(m) drop in OIS. In all the above experiments, we verified that immortalized HEC, not expressing the MEK:ER oncogene, did not display any alterations in senescence, mitochondrial calcium levels and Δψ(m) in response to 4OHT treatment ( Supplementary Fig. 7 ). 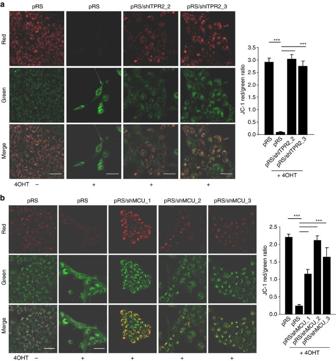Figure 6: Mitochondrial calcium accumulation during OIS provokes a drop in the mitochondrial potential. (a) HEC–TM cells were infected with a control empty vector (pRS) or with ITPR2-targeting shRNA retroviral vectors. After seeding they were treated for 3 days with 4OHT. Four days later, JC-1 probe was added and live fluorescence recorded and quantified. JC-1 red/green ratio was calculated to follow Δψ(m) (b) HEC–TM cells were infected with a control (ctrl) or with ITPR2-targeting shRNA retroviral vectors. They were next processed as described in (a) to measure Δψ(m) in the various conditions. Six to 12 fields were analyzed for each condition. Scale bar, 50 μM. Images shown are representative of experiments performed at least twice. Graphs are presented with s.e.m. as errors bars.P-values were determined using the studentt-test. *P<0.05; **P<0.01; ***P<0.001. Figure 6: Mitochondrial calcium accumulation during OIS provokes a drop in the mitochondrial potential. ( a ) HEC–TM cells were infected with a control empty vector (pRS) or with ITPR2-targeting shRNA retroviral vectors. After seeding they were treated for 3 days with 4OHT. Four days later, JC-1 probe was added and live fluorescence recorded and quantified. JC-1 red/green ratio was calculated to follow Δψ(m) ( b ) HEC–TM cells were infected with a control (ctrl) or with ITPR2-targeting shRNA retroviral vectors. They were next processed as described in ( a ) to measure Δψ(m) in the various conditions. Six to 12 fields were analyzed for each condition. Scale bar, 50 μM. Images shown are representative of experiments performed at least twice. Graphs are presented with s.e.m. as errors bars. P -values were determined using the student t -test. * P <0.05; ** P <0.01; *** P <0.001. 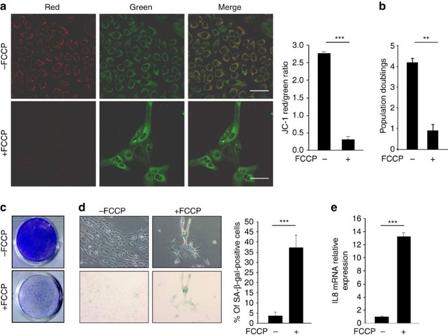Figure 7: Mitochondrial depolarization induces premature senescence. HEC–TM cells were seeded at the same density and treated or not with 300 nM FCCP for 4 days. The following day, cells were analyzed. (a) Cells were incubated with JC-1 probe and live fluorescence (Em 500–560 nm=green, and Em 590–650 nm=red) was recorded and quantified. JC-1 red/green ratio was calculated to evaluate Δψ(m) (n>10 fields). (b) Cells were counted and the number of population doublings was calculated. (c) Cells were paraformaldehyde fixed and crystal violet stained to monitor cell growth. (d) Cells were fixed and SA-β-Gal staining performed. Mean±s.d. shown. (e) RNA were extracted and RT–qPCR against IL8 senescence marker performed. Results are normalized to β-actin levels. Experiments were performed in triplicate, and results displayed are representative of experiments performed at least twice. Scale bar, 50 μM. Graphs are presented with s.e.m. as errors bars, and the studentt-test was used to determine theP-value. **P<0.01; ***P<0.001. Full size image Figure 7: Mitochondrial depolarization induces premature senescence. HEC–TM cells were seeded at the same density and treated or not with 300 nM FCCP for 4 days. The following day, cells were analyzed. ( a ) Cells were incubated with JC-1 probe and live fluorescence (Em 500–560 nm=green, and Em 590–650 nm=red) was recorded and quantified. JC-1 red/green ratio was calculated to evaluate Δψ(m) ( n >10 fields). ( b ) Cells were counted and the number of population doublings was calculated. ( c ) Cells were paraformaldehyde fixed and crystal violet stained to monitor cell growth. ( d ) Cells were fixed and SA-β-Gal staining performed. Mean±s.d. shown. ( e ) RNA were extracted and RT–qPCR against IL8 senescence marker performed. Results are normalized to β-actin levels. Experiments were performed in triplicate, and results displayed are representative of experiments performed at least twice. Scale bar, 50 μM. Graphs are presented with s.e.m. as errors bars, and the student t -test was used to determine the P -value. ** P <0.01; *** P <0.001. Full size image Mitochondrial potential drop leads to ROS production Mitochondrial calcium accumulation and mitochondrial depolarization are known to generate ROS, which are OIS mediators [28] , [29] . First we analyzed whether senescence was induced by oncogenic stress through ITPR2 involved ROS production. We observed an ROS increase in response to oncogenic stress in an ITPR2-dependent manner ( Fig. 8a ). Accordingly, we also observed a rise in ROS production during IP 3 - or FCCP-induced premature senescence ( Supplementary Fig. 8 ). Further supporting a role of ROS in mediating oncogenic stress/mitochondrial calcium accumulation-induced senescence, treatment with the anti-oxidant GSH resulted in OIS escape ( Fig. 8b ). 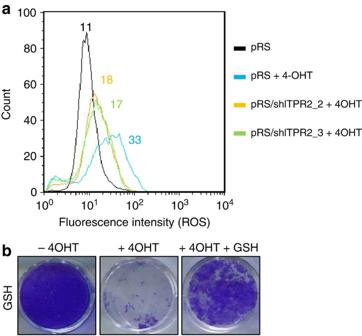Figure 8: ITPR2 activity regulates OIS through ROS production. (a) HEC–TM cells expressing or not ITPR2-directed shRNA were treated with 4OHT for 3 days. Two days later, cells were incubated with H2DCF-DA (30 min; 3 μM) and their ROS contents analyzed by FACS. (b) HEC–TM cells were treated with 4OHT for 3 days and GSH at 0.05 mM for 3 days. Figure 8: ITPR2 activity regulates OIS through ROS production. ( a ) HEC–TM cells expressing or not ITPR2-directed shRNA were treated with 4OHT for 3 days. Two days later, cells were incubated with H2DCF-DA (30 min; 3 μM) and their ROS contents analyzed by FACS. ( b ) HEC–TM cells were treated with 4OHT for 3 days and GSH at 0.05 mM for 3 days. Full size image Mitochondrial calcium participates in replicative senescence The above results were generated in the context of OIS, we next wanted to assess whether similar redistribution of calcium occurs during replicative senescence, a senescence induced by short telomeres and a DNA damage-like response, and not based on oncogenic stress. To this end, we used WI38 human fibroblasts [30] ( Supplementary Fig. 8a,b ). In accordance with OIS, replicative senescent fibroblasts were also found to display mitochondrial calcium accumulation ( Supplementary Fig. 9c,d ) and a Δψ(m) drop ( Supplementary Fig. 9e,f ). Importantly, MCU and ITPR2 knockdown inhibited these alterations during replicative senescence ( Supplementary Fig. 9g ) and delayed senescence ( Supplementary Fig. 9h,i ). Together, these data support a major role of calcium signalling and mitochondrial activity alterations during replicative senescence, suggesting that calcium displacement and ensuing consequences are general markers and actors of senescence. Using a loss-of-function genetic screen, we identified ITPR2 and MCU, two calcium channels whose depletion allowed OIS bypass. This identification has revealed a major role of calcium movement and mitochondrial calcium accumulation in the regulation of OIS. Importantly, the participation of these channels and mitochondrial calcium accumulation was also observed during replicative senescence. Overall, our results unveil a novel signalling pathway involving increased mitochondrial calcium uptake inducing OIS. In this study, we mainly investigated the role of mitochondrial calcium accumulation on senescence, following its release from the ER through ITPR2. The rationale for studying this was— calcium release by the ER can be transferred to the mitochondria [19] where calcium might exert deleterious effects (that is, apoptosis) [25] , [26] — and an shRNA directed against MCU, a transporter allowing mitochondrial calcium entry, was isolated during the genetic screen as potentially allowing OIS escape. The data accumulated confirm a prosenescent role of mitochondrial calcium accumulation. Indeed, the calcium accumulated in senescent cells (OIS, replicative senescence, induced by IP3) and its decrease by MCU knockdown results in senescence escape. ITPR channels are known regulators of other responses such as ER stress, autophagy and apoptosis [31] , [32] , [33] , [34] , [35] , [36] , [37] . The effect of ITPR2 on senescence did not appear to be linked to its role in ER stress ( Supplementary Fig. 10a ) or apoptosis ( Supplementary Fig. 10b ), as both of these remained unchanged during OIS. Autophagy, as described by others [38] , is modified during OIS, and this is partly reverted in ITPR2-knockdown cells ( Supplementary Fig. 10c ). Further studies will be required to determine a link between ITPR2, calcium and autophagy during senescence. The mitochondrial calcium accumulation observed during OIS or replicative senescence resulted in a decrease of the Δψ(m) and subsequent ROS production. Interestingly, decrease of the Δψ(m) is observed in senescent cells, in aging and in response to oncogenic stress [39] , [40] , [41] , [42] . Nevertheless, the mechanisms responsible for the deregulation of mitochondrial activity in stress-induced senescent cells are not known. Our data support the view that accumulation of mitochondrial calcium is responsible for the Δψ(m) drop induced during replicative or oncogene-induced senescence. In addition, we observe that decreased Δψ(m) leads to ROS production that according to our results, has an impact on senescence. It is also possible that other processes affected by mitochondrial activity alterations, such as decreased ATP production during senescence, participate in senescence regulation [30] , [41] , [43] , [44] , [45] . We have recently reported that the decreased ATP levels during OIS in the same model correlated with decreased glucose entry and metabolism [46] . In light of our results, we speculate that the mitochondrial alterations we observed also contribute to decrease ATP levels. In conclusion, our results outline a new pathway, controlled by ITPR2, but also by other ITPR and MCU calcium channels causing mitochondrial calcium accumulation, which decreases mitochondrial activity, and induces ROS accumulation and senescence. Our results offer new perspectives for understanding and developing new tools to manipulate senescence and its related disorders. Cell culture HECs (Lonza) were cultured in mammary epithelial cell growth medium (Promocell) supplemented with penicillin/streptomycin 100 U ml −1 (Life Technologies). Virus-packaging GP293 cells (Clontech) and human fibroblasts WI38 cells (ATCC) were cultured in Dulbecco’s modified Eagle’s medium (DMEM, Life Technologies) supplemented with 10% foetal bovine serum (Life Technologies) and penicillin/streptomycin 100 U ml −1 (Life Technologies). The cells were maintained at 37 °C under a 5% CO 2 atmosphere. Vectors and gene transfer Retrovirus pRetroSuperpuro (pRS) encoding shRNAs directed against ITPR2 and MCU were constructed by subcloning oligonucleotides targeting the following sequences: sh2 ITPR2 5′-GAGAAATGTTAGAGAAGAA-3′, sh3 ITPR2 5′-CAGAAAACTACTAGAGAAA-3′, sh1 MCU 5′-CGGCTTACCTGGTGGGAAT-3′, sh2 MCU 5′-AGGCAGAAATGGACCTTAA-3′, sh3 MCU 5′- GTTTTGACCTAGAGAAATA as described in Brummelkamp et al. [47] Mitochondrial calcium fluorescent genetic reporter ‘mito-GCaMP2’ was extracted by digestion with StuI-HindIII from pCDN3.1 vector [22] and cloned EcoRV-HindIII into pLNCX2 retroviral vector (Clontech). The plasmid pNLCΔMEK1 (ΔN3, S218E, S222D):ER was used to transfer the MEK oncogene. PEI reagent (Euromedex) was used according to the manufacturer’s recommendations to transfect GP293 cells with the indicated vector. Two days after transfection, the virus-containing supernatant was mixed with fresh medium (1/2) and hexadimethrine bromide at 8 μg ml −1 (Sigma) and used to infect target cells. Infected HECs were selected with G418 (Life Technologies) at 100 μg ml −1 and/or puromycin (InvivoGen) at 500 ng ml −1 . Knockdown of ITPR1 or ITPR3 was performed using Mission Lentiviral Transduction particles targeting ITPR1 (NM_002222) or ITPR3 (NM_002224) (or Green Fluroscent Protein as control) purchased from Sigma-Aldrich (clone ID TRCN0000061244 and TRCN0000061326). Chemicals 4OHT (Sigma) was used daily for 3 days at 250 nM. FCCP (sc-203578, Santa Cruz) was used daily at 300 nM, 236-Tri-O-Butyryl-myo-Inositol-145-Trisphosphate-Hexakis(acetoxymethyl) Ester, IP 3 -AM (Sichem) was used at a final concentration of 5 μM. 10 mM Ru360 (Sigma) was used to inhibit MCU. Reduced glutathione (GSH) (Sigma) was used at a concentration of 0.05 mM. ROS quantification Cellular ROS contents were measured by incubating cells with 3 μM H 2 DCF-DA probe for 30 min. The cells were washed in phosphate-buffered saline (PBS) (1 × ) buffer, trypsinised, washed again and resuspended in 500 μl PBS. ROS levels were analyzed by Fluorescence Activated Cell Sorting on a FACSCalibur flow cytometer, with 10,000 events recorded. The final data were analyzed using the Flow Jo 7.5.5 software. SA-β-Gal analysis and growth assays Cells were seeded into six-well plates. Briefly, for growth assays, cells were washed in PBS, fixed for 15 min in 3% formaldehyde and then coloured with a crystal violet solution. For SA-β-gal assay, cells were washed twice in PBS, fixed for 5 min (room temperature) in 2%formaldehyde/0.2% glutaraldehyde, washed twice in PBS, and incubated overnight at 37 °C (no CO2) with a fresh SA-β-Gal stain solution as previously described in Augert et al. [30] Immunoblotting Protein extracts were resolved by SDS-polyacrylamide gel electrophoresis and transferred to 0.45 μm nitrocellulose membrane (BioRad). Membranes were blocked in PBS containing 5% nonfat milk, 0.05% Tween 20. They were then probed overnight at 4 °C with the appropriate antibodies and dilutions. The secondary antibodies were either a peroxidase-conjugated donkey antirabbit immunoglobulin G or a peroxidase-conjugated goat antimouse immunoglobulin G (Jackson ImmunoResearch Laboratories, 1:5,000). Peroxidase activity was revealed using an enhanced chemiluminescence kit (GE healthcare). The primary antibodies used were: anti-phosphoERK (1:1,000, 9101, Cell Signalling), anti-phospho-histone3Ser10 (1:1,000, ab14955, Abcam), anti-active caspase 3 (1:250, ab 32042, Abcam), anti-LC3 (1:7,500, PM036, MBL) and anti-tubulin (1:5,000, T6199, Sigma). Reverse transcription and real-time quantitative PCR Total RNA were extracted based on a phenol-chloroform protocol, using TriReagent (Sigma-Aldrich) and PhaseLockGel tubes (Eppendorf). 2 μg of total RNA was retro-transcribed into complementary DNA (cDNA) using The First-Strand cDNA Synthesis Kit (GE Healthcare, Chalfont St Giles, UK) according to the manufacturer’s instructions. A 1:60 dilution of this RT reaction mixture was used as the cDNA template for qPCR. TaqMan qPCR was carried out on a LightCycler 2.0 System (Roche Applied Science). The final qPCR mixture was composed of the LightCycler TaqMan mix (dilution 1:5) (Roche), 200 nM of primers, the Universal Probe Library probe (100 nM) for the gene of interest (TaqMan Gene Expression Assays (primers/probe), Life Technologies) added up with 1.67 μl of cDNA template. All reactions were performed in triplicate. The relative amount of mRNA was calculated by the comparative Cp method following normalization against β-actin. The primers and probes used are listed in the Supplementary Table 2 . Confocal microscopy Samples were analyzed with a Zeiss LSM 780 NLO confocal microscope using a × 63 oil or a × 40 oil objective. During imaging, live cells were maintained at 37 °C in the microscope's environmental chamber. Image acquisition was carried out with the same gain, amplification, and exposure time between each experimental condition and the corresponding control. Images were captured using the Zen software and were then processed (cropping, addition of scale bars) using NIH ImageJ. Fluorescence intensity was measured with the ImageJ software. In each 8 bit image, fluorescence intensity above an automatic threshold was measured and if necessary, the corresponding area was also recorded. Calcium imaging and mitochondrial labelling Cells were plated in glass-bottom dishes (ThermoScientific-Nunc). Cells were transduced with a modified baculovirus coding a mitochondrial protein fused to a RFP according to the manufacturer’s recommendations (CellLight Mitochondria-RFP, BacMam 2.0, C10505, Life Technologies). Sixteen hours post-transduction, Oregon Green488 dye (O-6147, Molecular Probes) was used to visualize any change in calcium localization in the cytoplasmic compartment. Cells were washed three times with 1 ml of HBSS without calcium (Life Technologies), treated with Oregon Green488 dye at 2 nM for 30 min at 37 °C and washed twice with HBSS without calcium. Live cells were analyzed using confocal microscopy (Ex 561 nm/Em535–690 m). Alternatively, cells were transduced with a genetically encoded mitochondrially targeted calcium indicator. Following selection with G418, cells were seeded in glass-bottom dishes and treated with 4OHT, IP 3 -AM or FCCP as indicated. Fluorescence (Ex 488 nm/Em 500–570 nm) was investigated in live cells using Zeiss LSM 780 confocal microscope. Fluorescence intensity was quantified (ImageJ). Results were calculated by dividing the mean pixel intensity by the area of the measured spot. In short-term analysis, fluorescence was recorded every 1.5 s using a Zeiss LSM 780 confocal microscope. The duration of the change in mitochondrial calcium change at a region-of-interest (ROI) was calculated as the average of each ROI. Permeant-IP 3 was injected after 1 min of measurement at a final concentration of 5 μM. Results are shown as (F1-F0)/F0, where F0 is the mean of the intensities from 10 s to 50 s. Mitochondrial membrane potential Cells were plated in glass-bottom dishes (ThermoScientific-Nunc). To measure Δψ(m), cells were washed three times with 1 ml of HBSS without calcium, incubated with 10 μM Rhodamine 123 (R-302, Life Technologies) for 30 min, and washed again extensively before analysis by confocal microscopy (Ex 514 nm/Em520–660 nm). Alternatively, a ratiometric JC-1 probe (M34152, Life technologies) was used to discriminate energized and de-energized mitochondria. Fluorescence emission shift from green (530 nm) to red (590 nm) occurs when the dye is concentrated. As red fluorescent aggregates in areas with high potential membrane, mitochondrial depolarization is indicated by decreased red/green fluorescence intensity ratio. Cells were washed, incubated 10 min at 37 °C with 2 μM JC-1, washed extensively and fluorescence emission was recorded using an LSM 780 Zeiss confocal microscope (Ex 488 nm/Em 500–560 nm/590–650 nm). ER-mito contact sites A Z-stack of optical sections was captured using a Zeiss LSM 780 confocal microscope with an Apochromat 63 × /1.40 oil objective (0.720 μM slice thickness, 30 Z sections collected at 0.360 μM intervals). Nuclei were labelled with Hoechst, ER were labelled with anti-calnexin (C5C9, 2679, Cell Signalling), and MitoProfile Total OXPHOS Human Antibody Cocktail (ab110411, Abcam) was used to label mitochondria. Colocalisation between ER and mitochondria was quantified using Manders’ overlap coefficient. Statistics Graphs are presented with s.e.m. as errors bars, unless stated otherwise, and the student t -test was used to determine the P -value. * P <0.05; ** P <0.01; *** P <0.001 unless specified otherwise in the figure legends. How to cite this article: Wiel, C. et al. Endoplasmic reticulum calcium release though ITPR2 channels leads to mitochondrial calcium accumulation and senescence. Nat. Commun. 5:3792 doi: 10.1038/ncomms4792 (2014).